Sex differences in oncogenic mutational processes 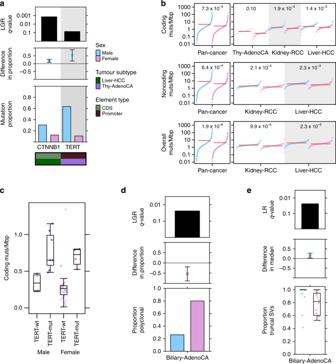Fig. 1: Sex-biases in mutation frequency of driver genes, SNV density and tumour evolution. aFrom top to bottom, each plot shows the logistic regressionq-value for the sex effect; difference in proportion of mutated samples between the sexes with blue denoting male-dominated bias; and mutation proportion for each gene. Covariate bars indicate mutation context and tumour subtype of interest.bThe burden of somatic SNVs for coding, non-coding and overall mutation load. Linear regressionq-values are shown.cCoding mutation load for thyroid adenocarcinoma samples compared by sex and presence or absence ofTERTpromoter mutations.dThe proportion of polyclonal samples andethe proportion of truncal structural variants in biliary cancer. Tukey boxplots are shown with the box indicating quartiles and the whiskers drawn at the lowest and highest points within 1.5 interquartile range of the lower and upper quartiles, respectively. Error bars show the 95% confidence interval for the difference in proportions or medians between the sexes. Sex differences have been observed in multiple facets of cancer epidemiology, treatment and biology, and in most cancers outside the sex organs. Efforts to link these clinical differences to specific molecular features have focused on somatic mutations within the coding regions of the genome. Here we report a pan-cancer analysis of sex differences in whole genomes of 1983 tumours of 28 subtypes as part of the ICGC/TCGA Pan-Cancer Analysis of Whole Genomes (PCAWG) Consortium. We both confirm the results of exome studies, and also uncover previously undescribed sex differences. These include sex-biases in coding and non-coding cancer drivers, mutation prevalence and strikingly, in mutational signatures related to underlying mutational processes. These results underline the pervasiveness of molecular sex differences and strengthen the call for increased consideration of sex in molecular cancer research. Sex disparities in cancer epidemiology include an increased overall cancer risk in males corresponding with higher incidence in most tumour types, even after adjusting for known risk factors [1] , [2] . Cancer mortality is also higher in males, due in part to better survival for female patients in many cancer types, including those of the colon and head and neck [3] . Interestingly, female colorectal cancer patients respond better to surgery [4] and adjuvant chemotherapy, though this is partially due to biases in tumour location and microsatellite instability [5] . Similarly, premenopausal female nasopharyngeal cancer patients have improved survival regardless of tumour stage, radiation or chemotherapy regimen [6] . There is a growing body of evidence for sex differences in cancer genomics [7] , [8] , [9] , [10] , [11] , [12] , but their molecular origins and clinical implications remain largely elusive. Previous studies have mostly focused on protein coding regions, leaving the vast majority of the genome unexplored. We hypothesise that there are uncharacterised sex differences in the non-coding regions of the genome. Using data from the Pan-cancer Analysis of Whole Genomes (PCAWG) project [13] , we perform a survey of sex-biased mutations in 1983 samples (1213 male, 770 female) from 28 tumour subtypes, excluding those of the sex organs (Supplementary Data 1 ). The PCAWG Consortium aggregated whole-genome sequencing data generated by the ICGC and TCGA projects. These data were re-analysed with standardised, high-accuracy pipelines to align to the human genome (reference build hs37d5). Our study leverages mutation calls generated by PCAWG working groups [13] , [14] , [15] , [16] to identify molecular associations with sex. We exclude the X and Y chromosomes to focus on autosomal sex differences in cancers affecting both men and women, but there are known to be significant X-chromosome mutational differences between tumours arising in men and women [8] . Our analysis reveals sex differences in specific genes and in genome-wide phenomena including mutation signature activity. These sex-biases occur not only at the pan-cancer level across all 1983 tumours, but also in individual tumour subtypes. Sex-biases in driver genes, mutation load and tumour evolution We began by investigating sex differences in driver gene mutation frequencies, focusing on 165 coding and nine non-coding mutation events [14] (Supplementary Data 2 ). We used proportion tests to identify candidate sex-biased events with a false discovery rate (FDR) threshold of 10%. These putative sex-biased events were modelled using logistic regression (LGR) to adjust for tumour subtype-specific variables (model descriptions and variable breakdown in Supplementary Data 1 ). Finally, we vetted these sex-biased events in two ways: we assessed the impact of covariate imbalances in the data using repeated down-sampling analysis; we also implemented extended regression models to adjust for additional variables like stage or grade, which were only available for a greatly reduced subset of the data (see “Methods” section). We confirmed that all sex-biases remained significant under this additional scrutiny. This statistical framework formed the basis for our analysis of all genomic features. Tumour subtype-specific sex-biased driver mutations included CTNNB1 mutation frequency in liver hepatocellular cancer (Liver-HCC), with more male-derived samples harbouring CTNNB1 mutations: (male: 31%, female: 13%, 95% CI: 8.1–28%, prop-test q = 0.048, LGR q = 1.4 × 10 −3 , Fig. 1a , Supplementary Fig. 1 ). This mirrors our previous finding of sex-biased CTNNB1 mutation frequency in liver cancer from TCGA exome sequencing data, with similar effect sizes (male: 33% vs. female: 12% [11] ). We also identified a large sex-disparity in a non-coding driver event in thyroid cancer (Thy-AdenoCA): TERT promoter mutations were observed in 64% of male-derived samples compared with only 11% of female-derived samples (95% CI: 17–89%, prop-test q = 6.9 × 10 −3 , LGR q = 0.074, Fig. 1a , Supplementary Fig. 1 ), again supporting a previous finding [17] . We did not find pathogenic germline variants in TERT or CTNNB1 that might bias the detection of sex-associated somatic mutations in these genes. Other putative sex-biased events were detected, but were either not statistically significant after multivariate adjustment at present sample sizes (Supplementary Data 2 ), or were attributed to over-represented tumour subtypes (Supplementary Fig. 2 ). Fig. 1: Sex-biases in mutation frequency of driver genes, SNV density and tumour evolution. a From top to bottom, each plot shows the logistic regression q -value for the sex effect; difference in proportion of mutated samples between the sexes with blue denoting male-dominated bias; and mutation proportion for each gene. Covariate bars indicate mutation context and tumour subtype of interest. b The burden of somatic SNVs for coding, non-coding and overall mutation load. Linear regression q -values are shown. c Coding mutation load for thyroid adenocarcinoma samples compared by sex and presence or absence of TERT promoter mutations. d The proportion of polyclonal samples and e the proportion of truncal structural variants in biliary cancer. Tukey boxplots are shown with the box indicating quartiles and the whiskers drawn at the lowest and highest points within 1.5 interquartile range of the lower and upper quartiles, respectively. Error bars show the 95% confidence interval for the difference in proportions or medians between the sexes. Full size image Our previous work [11] found sex-biased mutation density across a number of tumour subtypes, including cancers of the liver, kidney and skin. We therefore investigated mutation density here to identify tumour subtypes where the cancer genomes of one sex accumulate more somatic single nucleotide variants (SNVs) than those of the other sex. Returning to our statistical framework, we first used Mann–Whitney U -tests to identify putative sex-biases, and then applied multivariate linear regression (LNR) on Box–Cox transformed mutation load to adjust for possible confounders. The Box–Cox transformation applies a power function to modify the shape of a variable’s distribution to better approximate a normal distribution. It preserves monotonicity and is often applied to make data more suitable for regression analysis (see “Methods” section). We also compared the total number of somatic SNVs and further divided mutations by coding and non-coding SNVs to determine whether sex-biases may be influenced by specific genomic contexts. Across all pan-cancer samples, we identified higher mutation prevalence in male-derived samples in all three contexts (coding LNR q = 7.3 × 10 −4 , non-coding LNR q = 6.4 × 10 −4 , overall LNR q = 1.9 × 10 −6 ; Supplementary Data 3 ). These sex-biases remained significant even after adjusting for tumour subtype, ancestry and age in multivariate analysis, and after evaluating the effects of imbalanced tumour subtype and sex sample sizes (Fig. 1b, left; Supplementary Figs. 2 , 3 ). We investigated somatic SNV burden in each of the 23 individual tumour subtypes with at least 15 samples ( n male + n female ≥ 15), applying the same statistical approach using tumour subtype-specific models (Supplementary Data 1 ). We found sex-biased mutation load in three tumour subtypes (Fig. 1b , right), with trending higher male coding mutation load in thyroid cancer (difference in location = 0.26 mut/Mbp, 95% CI = 0.12–0.43 mut/Mbp, U -test q = 0.028, LNR q = 0.10), and higher male SNV load in hepatocellular cancer and kidney renal cell cancer (Kidney-RCC) for all three genomic contexts (Supplementary Data 3 ). We compared the group rank differences of coding and non-coding mutation load between the sexes and found that in renal cell cancer, the differences were similar at 0.40 mut/Mbp for non-coding mutations and 0.37 mut/Mbp for coding mutations. In hepatocellular cancer however, the median sex-difference in non-coding mutation load was higher than the difference in coding mutation load (non-coding difference = 0.84 mut/Mbp vs. coding difference = 0.53 mut/Mbp). There was a similar effect for pan-cancer mutations (non-coding difference = 0.60 mut/Mbp vs. coding difference = 0.41 mut/Mbp) suggesting mutation context may have a role in sex-biased SNVs in some tumour subtypes. On detecting sex differences in both the mutation frequency of specific drivers as well as SNV density in the same tumour subtypes, we asked whether one may bias the other. For instance, higher CTNNB1 mutation frequency in male-derived tumours may simply be due to more mutations occurring in those same samples. We therefore looked for associations between SNV burden with CTNNB1 mutation in hepatocellular cancer, and with TERT promoter mutation in thyroid cancer. We did not find a significant association between SNV burden and CTNNB1 mutation in hepatocellular cancer. In thyroid cancer however, TERT promoter mutation was associated with increased overall mutation burden (median TERT-wt = 0.32 mut/Mbp vs. median TERT-mut = 0.82 mut/Mbp, U -test p = 7.9 × 10 −8 ). We further confirmed the association using a linear regression model (linear regression p TERT = 2.4 × 10 −5 , p sex = 0.37, Fig. 1c ). To assess whether the sex-bias in TERT promoter mutation frequency might be due to sex-biased accumulation of SNVs, we examined tumour-matched mutation timing data generated by the PCAWG consortium [15] . We found that of eleven polyclonal samples with TERT promoter mutations, nine of these were earlier occurring truncal events. We continued investigating whether sex-biased driver mutations might occur at different stages of tumour evolution between men and women and examined tumour subclonal architecture. Focusing only on thyroid tumours with TERT promoter mutations and liver tumours with CTNNB1 mutations, we compared the proportions of polyclonal vs. monoclonal tumours between the sexes (Supplementary Fig. 4 ). We did not find sex-biased polyclonality in TERT promoter-mutated tumours, but did detect a putative bias in the proportion of polyclonal CTNNB1 -mutated tumours (80% of male-derived tumours are polyclonal vs. 46% of female-derived tumours, 95% CI = −0.019–0.70, prop-test p = 0.039). We therefore accounted for polyclonality when comparing the timings of the mutations in these driver events. On subsequently examining the frequency of clonal vs. subclonal driver mutation events between the sexes, we found that while there were differences in the proportions of truncal mutations (e.g. 100% of TERT promoter mutations were truncal events in male-derived vs. 50% truncal events in female-derived thyroid cancer patients), no comparisons were statistically significant. We expanded our clonality analysis to perform a general survey of clonal structure and mutation timing across all tumour subtypes and mutations (Supplementary Data 4 ). We found that female-derived biliary adenocarcinoma (Biliary-AdenoCA) tumours were frequently polyclonal, whereas most male-derived tumours were monoclonal (26% male-derived samples are polyclonal vs. 80% female-derived, 95% CI = 19–88%, prop-test q = 0.063, LGR q = 0.026; Fig. 1d ). In addition, we found intriguing evidence suggesting there may be sex differences in the mutation timing of structural variants (SVs) in this tumour subtype. Structural variants in male-derived samples were more frequently truncal events than in female-derived samples (median male percent truncal SVs = 100% vs. median female = 82%, 95% CI = 0.9–32%, U -test q = 0.081, LNR q = 8.6 × 10 −3 ; Fig. 1e ). Though other comparisons did not reach our statistical significance threshold, we found some interesting trends that may merit future study, including in oesophageal cancer (Eso-AdenoCA) where SVs in female-derived samples were more frequently truncal events while SVs in male-derived samples occurred more frequently in subclones (median male percent truncal SVs = 55%, median female = 100%; Supplementary Fig. 5 ), and in medulloblastoma, where insertion-deletions (indels) were more frequently truncal events in female-derived samples than male (median male percent of truncal indels = 65%, median female proportion of truncal indels = 70%; Supplementary Fig. 6 ). Our analysis of sex differences in tumour evolution identified some sex-biased events and hint at putative sex-biases that should be further explored in future analyses. Sex-biases in genome instability and CNAs Next, we examined percent genome altered (PGA), which provides a summary of copy number aberration (CNA) load. A proxy for genome instability, PGA is a complementary measure of mutation density to somatic SNV burden. Although we did not find associations between sex and autosome-wide PGA, we observed sex-biases in the copy number burden for specific chromosomes (Fig. 2a ). In pan-cancer analysis, male-derived samples exhibited a slight but significant higher percent chromosome altered for chromosome 7 even after accounting for tumour subtype, ancestry and age (median male PGA-7 = 5.4%, median female PGA-7 = 0.37%, 95% CI = 9.4 × 10 −4 –2.4 × 10 −3 %, U -test q = 5.0 × 10 −3 , LNR q = 0.024; Supplementary Data 5 ). In individual tumour subtypes, we found sex-biased PGA in renal cell cancer (chromosomes 7 & 12) and hepatocellular cancer (chromosomes 1 & 16). On further scrutinising these sex-PGA associations using extended models, we found that grade was a likely confounder in renal cell cancer, though the sex effect after correcting for this variable was still trending (extended LNR q = 0.17). By looking at copy number gains and losses separately, we additionally identified chromosomes with sex-biases in the burden of copy number gains and losses (Supplementary Fig. 7 and Supplementary Data 5 ), including sex-biased percent copy gained on chromosomes 5, 8 and 17 in pan-cancer tumours. These biases in chromosome instability were robust to imbalanced sex sample sizes (Supplementary Fig. 8 ). Fig. 2: Sex-biases in percent chromosome altered are reflected in gene-specific events. a A summary of associations between sex and genome instability across tumour subtypes. Dot size shows difference in median percent genome altered or percent chromosome altered between the sexes. Dot colour shows direction of bias, with blue indicating higher instability in male-derived tumours and pink indicating higher instability in female-derived tumours. Background shading shows q -values from multivariate linear regression. Sex differences in CNAs for b pan-cancer, c kidney renal cell cancer, and d hepatocellular cancer. Each plot shows, from top to bottom: the q -value showing significance of sex from multivariate linear modelling with yellow/green points corresponding to 0.1 < q < 0.05, deep blue/red points corresponding to q < 0.05, and grey points indicating hits that were attributed to covariate sample size imbalances and rejected; the proportion of samples with aberration; the difference in proportion between male and female groups for copy number gain events; the same repeated for copy number loss events; and the copy number aberration (CNA) profile heatmap. The columns represent genes ordered by chromosome. Light blue and pink points represent data for male- and female-derived tumours respectively. Full size image We next compared CNA frequency on the gene level to identify specific genes lost or gained at sex-biased rates. Across all pan-cancer samples, we found 2,502 genes with sex-biased gains across 13 chromosomes (LGR q -value < 10%, Fig. 2b , Supplementary Data 6 , 7 , Supplementary Figs. 2 , 9 ), These genes were all more frequently gained in male-derived samples than female, with differences in copy number gain frequency up to 10% on chromosomes 7 and 8. Genes with male-dominated copy number gains include the oncogene MYC (male gain frequency = 37% vs. female gain frequency = 28%, 95% CI = 5.2–14%, prop-test q = 2.5 × 10 −3 , LGR q = 0.068). The driver CTNNB1 was also more frequently gained in male samples (male gain frequency = 8.9% vs. female gain frequency = 5.2%, 95% CI = 1.4–6.1%, prop-test q = 0.016, LGR q = 0.053). We did not find pan-cancer sex-biased copy number losses. We repeated this analysis for every tumour subtype independently and found sex-biased CNAs in renal cell and hepatocellular cancer (Supplementary Data 6 and 7 ). In renal cell cancer (Kidney-RCC), 1,986 sex-biased gains all occurred more frequently in male-derived samples, with differences in frequency up to 35% (Fig. 2c ). They spanned across chromosomes 7 and 12, agreeing with our finding of male-dominated genome instability in these chromosomes (Fig. 2a ; Supplementary Fig. 7 ). Using an extended renal cell cancer model accounting for grade, we obtained a high confidence set of 969 genes altered by sex-biased gains (extended model q < 0.1), with the remaining 1017 genes having a trending sex effect (extended model q < 0.17). In contrast to the male-dominated gains in pan-cancer and renal cell findings, we found higher female frequency of copy number losses in hepatocellular cancer (Fig. 2d ). We identified 2226 genes with higher copy number loss rates in female-derived samples. As observed in renal cell cancer some of these losses span whole chromosomes, in this case chromosomes 3 and 16. Extended modelling in Liver-HCC incorporating stage and grade resulted in a list of 1797 high confidence sex-biased genes (extended model q < 0.1). The concurrence between sex-biased PGA and gene-specific events in renal cell and hepatocellular cancer suggested that PGA could be used to guide identification of additional sex-biased CNAs on the gene level. We more closely examined regions of interest in tumour subtypes of that did not have sex-biased CNAs in our general CNA analysis, but did have putatively sex-biased genome instability ( U -test q < 0.2): biliary cancer, B-cell non-Hodgkin lymphoma (Lymph-BNHL), and chronic lymphocytic leukaemia (Lymph-CLL). We identified an additional 203 genes on the p-arm of chromosome 8 that were more frequently lost in female-derived biliary tumours (Supplementary Fig. 10 ). These copy number losses were 50% more common in female-derived tumours and affect genes such as DLC1 , a known tumour suppressor gene in hepatocellular cancer that is thought to have a similar role in gallbladder cancer [18] . Although we did not identify additional sex-biased CNAs in non-Hodgkin lymphoma, chronic lymphocytic leukaemia or melanoma, our sex-biased PGA results suggest these as regions of interest for future work. Sex-biases in mutational signatures We hypothesised that sex differences in mutation density and tumour evolution characteristics might be driven by sex differences in mutational processes. In addition to single base substitution (SBS) signatures, which have been well annotated and linked to tumour aetiology [19] , [20] , we also examined doublet base substitution (DBS) and small insertion-deletion (ID) signatures. Sex differences in a mutational signature could shine insight on molecular differences between the sexes. For each of 47 validated PCAWG SBS, 11 DBS and 17 ID signatures [16] , we performed a two-stage analysis. We first compared the proportions of signature-positive samples between the sexes; that is, we looked at the proportions of samples with any mutations attributed to the signature to determine whether there was a relationship between each signature and sex. Then, we focused on signature-positive samples and compared the percentage of mutations attributed to each signature between the sexes to assess relative signature activity. For both analyses we used univariate techniques to identify putative events, adjusted for additional variables using linear models with SNV density as a variable, and compared the distributions of attributed mutations with Kolmogorov–Smirnov tests. We also evaluated hits using the added scrutiny of down-sampling and extended regression models (see “Methods” section; Supplementary Figs. 11 , 12 ). At the pan-cancer level, we identified three signatures that occurred more frequently in one sex over the other (Fig. 3a ; Supplementary Data 8 ). SBS1 was more commonly detected in female-derived samples (88% of male-derived vs. 97% of female-derived, χ 2 -test q = 9.2 × 10 −10 , LGR q = 3.0 × 10 −6 ) and was also associated with higher signature activity in these samples (male median percent mutations attributed to SBS1 = 8.6%, female median = 10%, U -test q = 5.5 × 10 −3 , LNR q = 0.059). Conversely, signatures SBS17a and SBS17b were detected in a larger proportion of male-derived samples (16% of male-derived vs. 7.2% of female-derived). SBS1 is thought to be caused by deamination of 5-methylcytosine to thymine, resulting in base substitutions. Signatures SBS17a and SBS17b are of unknown aetiology. We also identified a sex-bias in indel signature ID5, which had higher activity in female-derived tumours (male median percent attributed mutations = 35%, female median = 38%, U -test q = 1.1 × 10 −3 , LNR q = 0.053). ID5 mutations are clock-like and may accumulate in normal cells. Both SBS1 and ID5 are correlated with age, but our multivariate model accounts for this variable and sex-bias remains significant. Fig. 3: Sex differences in mutational signatures related to mutational processes. Comparisons between proportions of signature-positive samples (top) and signature activity (bottom) for a pan-cancer comparisons, b liver hepatocellular cancer, and c B-cell non-Hodgkin lymphoma. FDR-adjusted q -values for multivariate logistic regression (top) and multivariate linear regression (bottom) shown only for significant comparisons. Blue shows male- and pink shows female-derived tumours. Tukey boxplots are shown with the box indicating quartiles and the whiskers drawn at the lowest and highest points within 1.5 interquartile range of the lower and upper quartiles, respectively. Full size image Since mutational processes are disease-specific, we repeated the mutational signatures analysis in each tumour subtype. We identified six sex-biased signatures in hepatocellular cancer (Fig. 3b ; Supplementary Data 8 ). We again detected a female-dominated bias in the proportion of SBS1-positive samples (58% of male-derived vs. 88% of female-derived, χ 2 -test q = 3.5 × 10 −5 , LGR q = 6.3 × 10 −5 ). We also detected a male-dominated bias in SBS16 (16% of male-derived vs. 2.2% of female-derived, χ 2 -test q = 9.8 × 10 −3 , LGR q = 0.011). A previous study [21] described this sex-biased signature and an association between more CTNNB1 mutations and higher activity of SBS16 in an independent dataset; these findings agree with what we report here for PCAWG data. There were also four sex-biased ID signatures in hepatocellular cancer: ID3 (94% of male-derived vs. 81% of female-derived, χ 2 -test q = 5.0 × 10 −3 , LGR q = 0.011), ID8 (93% of male-derived vs. 78% of female-derived, χ 2 -test q = 3.5 × 10 −3 , LGR q = 4.6 × 10 −3 ) and ID11 (17% of male-derived vs. 1.1% of female-derived, χ 2 -test q = 3.5 × 10 −3 , LGR q = 0.011) occurred more frequently in male-derived samples. ID3 is associated with tobacco smoke, and ID8 with double-stranded break repair. ID11 has unknown aetiology. Although ID1 was detected at similar rates between the sexes, a greater proportion of ID1-attributed mutations were found in female-derived than male-derived samples (male median percent mutations attributed to ID1 = 21%, female median = 27%, U -test q = 2.4 × 10 −6 , LR q = 1.0 × 10 −5 ). Using our extended hepatocellular model to further scrutinise these signatures, we found that all remained sex-biased after accounting for these variables except in ID3, where the effect was trending (extended model q -value = 0.12). Mutations associated with ID1 are thought to result from slippage during DNA replication and are associated with defective DNA mismatch repair, suggesting that while male- and female-derived tumours harbour defective DNA repair at similar rates, it is responsible for a larger proportion of mutations in female-derived tumours. Taken together, sex-biases in the aetiology underlying the molecular landscape of hepatocellular cancer begin to emerge. In this tumour subtype, spontaneous or enzymatic deamination of 5-methylcytosine to thymine and defective mismatch repair occur more frequently in female patients and are also responsible for more mutations. Conversely, tobacco smoking is more common in male patients though the number of mutations attributed to tobacco smoke is not different between the sexes; this leads to more tobacco-associated male hepatocellular tumours. In B-cell non-Hodgkin lymphoma, we identified significant differences in the proportions of SBS17a- and SBS17b-positive tumours (Fig. 3c; Supplementary Data 8 ). More male-derived samples had mutations associated with these signatures. There were also several intriguing sex differences in mutational signatures that did not meet our significance threshold. For instance in thyroid cancer, DBS2 accounts for a higher percentage of mutations in male-derived samples (male median percent mutations attributed to DBS2 = 50%, female median = 33%, Supplementary Data 8 ). The association of DBS2 with tobacco smoking suggests that future insight in this signature may provide molecular explanations for the sex-specific associations between smoking and thyroid cancer risk [22] . As the aetiologies of these mutational signatures become better known, we can better understand how underlying mutational processes lead to molecular sex-biases. We may also be able to discern environmental and lifestyle factors even in the absence of reported data, allowing us to better account for confounding factors. Finally, to ensure that our findings were not skewed by differences in sequencing quality, we checked for sex-biases in quality control (QC) metrics. These included comparing the coverage, read length, and overall quality summaries of both tumour and normal genomes. We mirrored our main analyses and used Mann–Whitney U -tests or χ 2 tests and linear modelling to check each QC metric. We did not find sex-biases in any QC metric in pan-cancer or tumour subtype analysis after multiple adjustment except in raw somatic mutation calling (SMC) coverage. SMC coverage was higher in male-derived samples in six tumour subtypes including thyroid cancer and oesophageal cancer, and was higher in female-derived samples in lung adenocarcinoma and B-cell non-Hodgkin lymphoma (Supplementary Data 9 and Supplementary Fig. 13 ). Although we do not find sex differences in comparing the SMC coverage pass/fail rates using a recommended minimum of 2.6 gigabases covered, it is prudent to consider sex-biased SMC in relation to our findings. Our analysis of whole-genome sequencing data from the PCAWG project uncovered sex differences in the largely unexplored non-coding autosomal genome. In addition to validating previously reported findings in a novel dataset, we present sex-biases in measures of non-coding mutation density, tumour evolution and mutation signatures. These sex-biases suggest differences in the origins and trajectories of tumours between men and women, and that they are influenced by different endogenous and environmental factors. Although many of our findings describe pan-cancer differences, we have also uncovered an intriguing glimpse into tumour subtype-specific differences in cancers such as those of the liver and kidney. These results should be taken within context of a number of caveats. As we use techniques like the Box–Cox transformation to make the data better suited for our statistical methods, there are likely characteristics that our models are unable to account for. An alternate approach using robust modelling may be better suited for future analyses. Secondly, the tumour subtype-specific results are bound by subtype sample size, and lack of annotation data restricts the ability to account for confounding variables. It is therefore important to consider these results within context of the multivariable models used, which do not directly capture characteristics such as tobacco smoking history. Many of our core multivariate regression models omit stage and grade due to a large number of missing values. We follow up this core regression with extended modelling as an additional level of scrutiny. Although these extended models do include stage or grade, they are run on a much smaller (up to 50%) subset of the data and there is a corresponding loss of statistical power. Finally, there are imbalances across covariate sample sizes, such as over-representation of some tumour types in pan-cancer analysis. We evaluated these imbalances using down-sampling analysis and rejected results that were biased by these imbalances. Nevertheless, pan-cancer analysis is dependent on the tumour subtypes included in the cohort and some findings may reflect subtype-specific trends rather than general characteristics across all cancers. Future increases in sample size and robust associated annotation will allow for the detection of smaller effects and the control of more confounders. Such large datasets are critical in validating the preliminary findings we have described in this study. Increasing the diversity of donors will also allow the study of intriguing cross-variable questions such as investigating whether sex differences are universal across races, or if there are race-specific sex differences. Our results are based on single region sequencing, which can bias the clonal reconstruction for these tumours. Future work sampling multiple regions will allow us to detect sex differences in more precise reconstructions at a greater resolution. We will also be able to leverage germline data to assess whether there are sex-biases in inherited variants that affect the variants we observe in somatic mutation profiles. Nevertheless, our analyses of driver genes and copy number alterations suggest functional impacts of genomic sex-biases on the transcriptome and tumorigenesis. By using signatures to distinguish between mutations attributed to lifestyle factors such as smoking history, we can better describe sex differences related to biological factors such as hormone activity. And despite low tumour subtype-specific sample numbers, our mutation timing and mutational signatures findings at both the pan-cancer and tumour-subtype level hint at underlying mutational processes that may give rise to molecular sex-biases. Combined with our previous work in whole-exome sequencing, we present a landscape of sex-biases in cancer genomics and mutational processes (Fig. 4 ). Fig. 4: The landscape of sex differences in cancer genomics. Summary of genomic features found to be sex-biased in pan-cancer analysis or in specific tumour subtypes. Results from both PCAWG and TCGA analyses are shown. Direction of sex-bias is shown in coloration denoting which sex has higher or more frequent aberration of the genomic feature. Top plot shows union of genes found to be involved in sex-biased CNAs. Starred indicate findings exclusively from exome sequencing data ( n = 7131), un-starred indicate findings from PCAWG data ( n = 1983), and double-starred indicate findings also described in other studies. Full size image It is becoming clear that sex differences occur across many mutation classes and the portrait of differences for each tumour subtype is a unique reflection of active mutational processes and tumour evolution. We have performed here a pan-cancer analysis of sex differences in whole-genome sequencing data and catalogued previously undescribed sex-biases. However, increased study of molecular sex differences in future large-scale sequencing efforts is needed to strengthen the findings we present here, to determine why men and women have molecularly different tumours, and to determine how this information can be leveraged to improve patient care. General statistical framework We only included non-sex-specific tumour subtypes in our analysis and focused on the autosome, excluding the sex chromosomes. Covariate data include genomically matched sex, age at diagnosis, and imputed ancestry. For each genomic feature of interest, we performed three stages of analysis. At stage one, we use non-parametric univariate tests (Pearson’s χ 2 proportion or Mann–Whitney U -test) first, followed by false discovery rate adjustment to identify putative sex-biases of interest ( q < 0.1). At stage two, we further investigate these putative sex-biases by using multivariate linear or logistic modelling to account for potential confounders using bespoke models for each tumour subtype. Confounders were included as independent variables in each model. Supplementary Data 1 describes the model variables for each tumour context, as well as detail on when analyses included multivariate modelling. Variables were included based on availability of data (<15% missing), sufficient variability (at least two levels) and collinearity. Discrete data were modelled using logistic regression. Continuous data were first transformed using the Box–Cox family and modelled using linear regression. The Box–Cox family of transformations is a formalised method to select a power transformation to better approximate a normal-like distribution and stabilise variance. We used the Yeo–Johnson extension to the Box–Cox transformation that allows for zeros and negative values [23] : 
    y_i^λ = {[              ( y_i + 1)^λ - 1/λ,                  if λ   0, y ≥ 0;                   log( y_i + 1),                  if λ = 0, y ≥ 0; - (  - y_i + 1)^2 - λ - 1/2 - λ,                  if λ   2, y < 0;              - log(  - y_i + 1),                  if λ = 2, y < 0 ]..
 FDR adjustment was performed for p -values for the sex variable significance estimate and an FDR threshold of 10% was used to determine statistical significance. For some tumour subtypes, the multivariate step is never performed because there are no univariate hits to evaluate. The third stage of analysis involves re-evaluating our stage two sex-biases with a battery of additional modelling: For pan-cancer findings, we evaluate the effect of unbalanced tumour subtype sample sizes by repeatedly and randomly down-sampling to the median subtype sample size with replacement ( n median = 48). For each down-sampled dataset, we record the difference between the male and female median/proportion, as well as the p -value from the relevant univariate test (Supplementary Fig. 2 ). We repeat this 10,000 times for each finding to generate distributions of male–female differences and p -values. We calculate a 95% confidence interval using the male–female difference distribution and reject findings where this confidence interval overlaps with 0. We also reject findings where the median down-sampled p -value is greater than the p = 0.05 threshold. For both pan-cancer and tumour subtype-specific findings, we evaluate the effect of unbalanced sexes when either female or male donors account for >60% of samples. We down-sample to the smaller number of samples with replacement and record the difference between the male and female median/proportion, as well as the p -value from the relevant univariate test (Supplementary Figs. 1 , 3 , 8 , 9 and 11 ). We repeat this 10,000 times for each finding to generate distributions of male–female differences and p -values. We calculate a 95% confidence interval using the male–female difference distribution and reject findings where this confidence interval overlaps with 0. We also reject findings where the median down-sampled p -value is greater than the p = 0.05 threshold. We present the median down-sampled p -values throughout Supplementary Data 2 – 8 . For tumour subtype-specific results, we also use extended models that incorporate additional variables such as tumour stage. Because this leads to up to 50% data loss, we only investigate a subset of results in this way. All extended modelling results are presented in Supplementary Data 2 – 8 . Specific details are provided for each analysis below. Driver event analysis We focused on driver events ( syn11639581 ) described by the PCAWG consortium [14] . Driver mutation data were binarized to indicate presence or absence of the driver event in each patient. For the first stage of our analysis, we compared proportions of mutated genes between the sexes using univariate proportion tests. A q -value threshold of 0.1 was used to select genes for further multivariate analysis in stage two using binary logistic regression. FDR correction was again applied and genes with significant pan-cancer sex terms were extracted from the models ( q -value < 0.1). Driver event analysis was performed separately for pan-cancer analysis and for each tumour subtype. Clonal structure and mutation timing analysis Subclonal structure and mutation timing calls [15] were downloaded from Synapse ( syn8532460 ). Subclonal structure data were binarized from number of subclonal clusters per sample to monoclonal (one cluster) or polyclonal (more than one cluster). The proportion of polyclonal samples was calculated per sex and compared in the first stage of analysis using proportion tests for both pan-cancer and tumour subtype analysis. The univariate p -values were FDR-adjusted across all tumour subtypes to identify putatively sex-biased clonal structure. These cases were further scrutinised in stage two using logistic regression. A multivariate q -value threshold of 0.1 was used to determine statistically significant sex-biased clonal structure. Mutation timing data classified SNVs, indels and SVs into clonal (truncal) or subclonal groups. The proportion of truncal variants was calculated for each mutation type ( \(\frac{{{\mathrm{Number}}\,{\mathrm{truncal}}\,{\mathrm{SNVs}}}}{{{\mathrm{Total}}\,{\mathrm{SNVs}}}}\) , etc) to obtain proportions of truncal SNVs, indels and SVs for each sample. These proportions were compared in stage one of analysis between the sexes using two-sided Mann–Whitney U -tests and univariate p -values were FDR-adjusted to identify putatively sex-biased mutation timing. In stage two, linear regression was used to adjust for confounding factors and a multivariate q -value threshold of 0.1 was used to determine statistically significant sex-biased mutation timing. The mutation timing analysis was performed separately for SNVs, indels and SVs. SNV density analysis Consensus SNV calls were downloaded from Synapse ( syn7357330 ). Overall SNV density per patient was calculated as the sum of SNVs across all genes on the autosomes and scaled to mutations/Mbp. Coding mutation prevalence only considers the coding regions of the genome, and non-coding prevalence only considers the non-coding regions. Mutation load was first compared between the sexes using Mann–Whitney U -tests for both pan-cancer and tumour-type specific analysis. Comparisons with U -test q -values meeting an FDR threshold of 10% were further analysed using linear regression to adjust for tumour subtype-specific variables. Mutation load analysis was performed separately for each mutation context, with pan-cancer and tumour subtype p -values adjusted together. Chromosome and genome instability analysis Consensus copy number data were obtained from Synapse ( syn8042988 ). Ploidy-adjusted calls were used to identify segments with copy number gains and losses. The number of bases in copy number gained or lost segments were summed per chromosome and divided by chromosome size to obtain percent chromosome gained and lost, respectively. All segments affected by any copy number aberration were also summed and treated in the same way to calculate percent chromosome altered. Percent copy number gained, lost and altered were also calculated over the autosomes. In stage one, genome and chromosome instability were compared in pan-cancer and tumour-subtype analysis using Mann–Whitney U -tests to identify putatively sex-biased chromosome and genome instability. In stage two, putatively sex-biased events were further analysed using linear regression modelling. Genome instability analysis was performed separately for each tumour subtype with FDR adjustment performed over percent copy gained, loss and altered comparisons together. 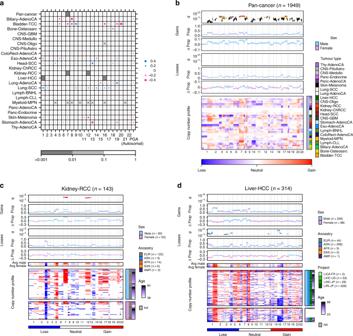Fig. 2: Sex-biases in percent chromosome altered are reflected in gene-specific events. aA summary of associations between sex and genome instability across tumour subtypes. Dot size shows difference in median percent genome altered or percent chromosome altered between the sexes. Dot colour shows direction of bias, with blue indicating higher instability in male-derived tumours and pink indicating higher instability in female-derived tumours. Background shading showsq-values from multivariate linear regression. Sex differences in CNAs forbpan-cancer,ckidney renal cell cancer, anddhepatocellular cancer. Each plot shows, from top to bottom: theq-value showing significance of sex from multivariate linear modelling with yellow/green points corresponding to 0.1 <q< 0.05, deep blue/red points corresponding toq< 0.05, and grey points indicating hits that were attributed to covariate sample size imbalances and rejected; the proportion of samples with aberration; the difference in proportion between male and female groups for copy number gain events; the same repeated for copy number loss events; and the copy number aberration (CNA) profile heatmap. The columns represent genes ordered by chromosome. Light blue and pink points represent data for male- and female-derived tumours respectively. Genome-spanning CNA analysis Consensus copy number data ( syn8042988 ) were processed to gain/neutral/loss calls per gene. For each gene, we compared the proportion of gains for each sex using proportion tests. For putative sex-biased genes that passed an FDR threshold of 10%, we followed up with multivariate logistic regression to adjust for tumour subtype-specific covariates (Supplementary Data 1 ). We repeated this analysis for copy number loss. This genome-spanning analysis was performed separately for losses and gains for each tumour subtype. Mutational signatures analysis The number of mutations attributed to each SBS ( syn11738669 ), DBS ( syn11738667 ) and ID ( syn11738668 ) signature [16] per sample was downloaded from Synapse. For each signature, we compared the proportion of samples with any mutations attributed to the signatures (“signature-positive”) using χ 2 -square tests to identify univariately significant sex-biases. Signatures with putative sex-biases were further analysed using logistic regression. We also compared the proportions of mutations attributed to each signature. The numbers of mutations per signature were divided by total number of mutations for each sample to obtain the proportion of mutations attributed to the signature. In the first stage of analysis, we used Mann–Whitney U -tests to compare these proportions of attributed mutations, and Kolmogorov–Smirnov tests to compare their distributions between the sexes. Putative sex-biased signatures were further analysed using linear regression after Box–Cox adjustment. In addition to tumour subtype-specific covariates, we included SNV density in all multivariate mutational signatures models to account for bias in calling more signatures in SNV-dense samples. Signatures that were not detected in a tumour subtype were omitted from analysis for that tumour subtype. We also used Kolmogorov–Smirnov tests to compare the distributions of attributed mutations and kept results where the sex-difference was significant or trending. 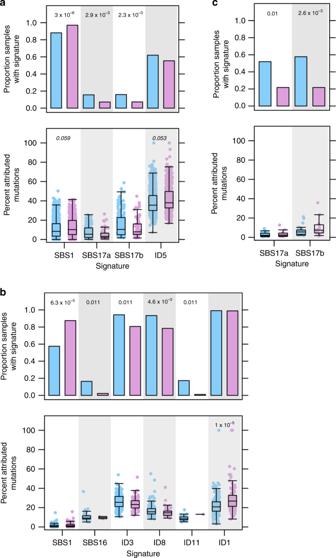Fig. 3: Sex differences in mutational signatures related to mutational processes. Comparisons between proportions of signature-positive samples (top) and signature activity (bottom) forapan-cancer comparisons,bliver hepatocellular cancer, andcB-cell non-Hodgkin lymphoma. FDR-adjustedq-values for multivariate logistic regression (top) and multivariate linear regression (bottom) shown only for significant comparisons. Blue shows male- and pink shows female-derived tumours. Tukey boxplots are shown with the box indicating quartiles and the whiskers drawn at the lowest and highest points within 1.5 interquartile range of the lower and upper quartiles, respectively. 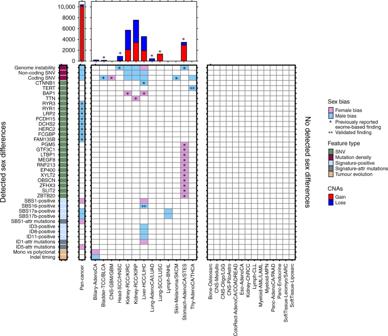Fig. 4: The landscape of sex differences in cancer genomics. Summary of genomic features found to be sex-biased in pan-cancer analysis or in specific tumour subtypes. Results from both PCAWG and TCGA analyses are shown. Direction of sex-bias is shown in coloration denoting which sex has higher or more frequent aberration of the genomic feature. Top plot shows union of genes found to be involved in sex-biased CNAs. Starred indicate findings exclusively from exome sequencing data (n= 7131), un-starred indicate findings from PCAWG data (n= 1983), and double-starred indicate findings also described in other studies. Reporting summary Further information on research design is available in the Nature Research Reporting Summary linked to this article.